The lifetime of the deviations from bulk behaviour in polymers confined at the nanoscale Monitoring the impact of annealing on the dynamic glass transition of nanometres-thick polymer layers provides new insights into the mechanisms behind the tremendous changes in the performance of macromolecular materials in close proximity to an interface. Here we present results revealing a correlation between deviations from bulk behaviour, manifesting in changes to the glass transition temperature, the reduction of dielectric strength and the growth of an irreversibly adsorbed layer (Guiselin brushes). The non-universal behaviour of polymers under confinement could be explained in terms of a dimensionless number given by the ratio between the timescale of adsorption and the annealing time. In particular, in the case of slow adsorption kinetics, such as for polystyrene on aluminium, deviations from bulk behaviour correspond to metastable states with an extremely long lifetime. The proximity of solid interfaces and free surfaces tremendously alters the behaviour of any material [1] , [2] , [3] , [4] , [5] . Polymers are particularly affected by these perturbations because of the higher conformational entropy introduced by monomer connectivity. As a consequence, in ultrathin polymer films (thickness <200 nm), parameters such as flow and intermolecular entanglements [6] , local chain mobility and glass transition temperature ( T g ) [2] , [7] , [8] , physical aging [9] , creep behaviour [3] , gas permeability [10] and crystallization kinetics [11] , [12] can differ substantially from their bulk values. Unexpectedly, deviations from bulk behaviour are also sensitive to the annealing conditions used during sample preparation. Although the reduction of mechanical stresses can be achieved even in the glassy state ( T < T g ), albeit after several months [13] , reproducible measurements of T g are expected only at thermodynamic equilibrium on annealing in the liquid state ( T > T g ), at times longer than the terminal relaxation (reptation) time, τ REP . The reptation model [14] predicts that polymer chains equilibrate at timescales on the order of τ REP , after completely disentangling from the tube induced by screening of neighbouring segments. Several experimental observations, however, seem to contradict this basic concept of polymer science [15] , [16] , [17] , [18] , [19] , [20] . Barbero and Steiner [18] probed the rheological properties of films of polystyrene (PS) thicker than 100 nm; their measurements revealed that immediately after film formation (spincasting), chains are trapped in non-equilibrium conformations conferring a reduced effective viscosity. Bulk-like values could be recovered only after severe annealing at timescales much longer than τ REP , for example, 145 h at T g +55 K were sufficient to equilibrate chains with a molecular weight ( M w )=113 kg mol −1 , whereas films of M w =665 kg mol −1 could not recover bulk viscosities after being annealed for more than 1 week. Similar trends were observed for the structural relaxation time, τ α , of poly(methyl methacrylate) (PMMA) and of poly(vinyl acetate) [17] . In samples kept below T g , the structural relaxation was faster by several orders of magnitude compared with bulk conditions, yet the separation between τ α of the film and its bulk value decreased during successive heating scans in the liquid state, without ever vanishing completely, for samples of poly(vinyl acetate). By selectively placing layers of dye-labelled PS (having a larger dielectric response) at different depths inside films of pristine PS, we verified that the perturbations of the local T g on annealing are restricted to molecules in direct contact with an adsorbing interface [21] . These observations suggest that changes in the properties of polymer chains at the nanoscale level related to interfacial interactions, have a finite lifetime and that the deviations from bulk behaviour correspond to metastable states, that is, polymer conformations associated with local and not global minima of the free energy. Unveiling the mechanisms behind the response of polymers on annealing has both scientific and practical significance. From the scientific point of view, understanding the nature of the mechanisms behind the evolution of T g in different annealing conditions could finally lead to a detailed understanding of the behaviour of macromolecules in confined geometries. Similarly, quantifying the timescale of the perturbations affecting the interfacial properties would improve the design of sensors, coatings, nanostructured and functional polymeric materials and other devices exploiting enhanced properties of polymers at the nanoscale level. In this work, we aimed to identify an experimentally accessible quantity to measure the lifetime of the deviations from bulk behaviour and conditions that would freeze the polymer chains in the desired conformations for a timescale much longer than those of interest for technological applications. Impact of chain immobilization on the dielectric function We began our investigation after noticing a striking similarity between the changes in structural (α−) relaxation on annealing and those during isothermal crystallization: in both cases, minor variations in the relaxation time are accompanied by large reductions of the dielectric strength Δ ɛ , that is, the amount of mobile chains involved in structural relaxation and thus in the glass transition [22] . This effect is reflected in the thickness dependence of the structural relaxation process, as probed by dielectric spectroscopy. Regardless of whether thinner films exhibit a higher or lower T g , the relaxation time remains unaltered down to thicknesses on the order of 20 nm, whereas Δ ɛ , which scales with the surface-to-volume ratio (inverse of the thickness), decreases even at hundreds of nanometers [23] . These trends suggested that keeping a polymer layer above T g would favour the adsorption of chains at the interface. In analogy with crystallization, in fact, adsorption requires mass transport towards an interface and the optimization of chain conformations to achieve the highest gain in free energy on densification [24] . Deviations from bulk behaviour would originate from those non-equilibrium conformations assumed in the adsorbed layer [25] , [26] and evolve during annealing with the same kinetics as the adsorption process. To test this hypothesis, we designed an experiment that enables us to monitor the evolution of metastable states through which ultrathin polymer layers go during annealing. The thickness of the layer adsorbed at the interface was quantified independently at different annealing times in the same experimental conditions. An analysis of polymer films of different thicknesses and molecular weights confirmed that the impact of annealing on the structural relaxation and on T g shows excellent correlation with the growth of an irreversibly adsorbed layer at the polymer/substrate interface. Our approach is based on measuring, in real time and isothermal conditions, the variation of the dielectric function of films previously 'equilibrated' during a preannealing step much longer than τ REP . Electrical capacitances were measured by applying an A/C electric field perpendicular to the surface of the films and measuring the current flow generated. Under these conditions, for non-polar systems ( ζ =Δ ɛ / ɛ ∞ ≪ 1, where ɛ ∞ is the value of the dielectric constant in the absence of molecular polarization), the electrical impedance of the whole film can be linearly expressed as the sum of the capacitance of the sublayers contributing to the dielectric signal. This procedure is justified by the observation that the molecular dynamics of the whole film corresponds to the dynamics averaged over the different sublayers [27] . With the goal of direct analysis of our data, we have chosen PS ( ζ ≈0.016), a polymer with a dielectric strength large enough to be determined precisely by an impedance analyser, but much smaller than its dielectric constant, which allowed us to avoid nonlinear convolutions. Following typical annealing protocols described in the literature, we monitored the changes in the relaxation spectra of the samples at T > T g , where the structural (α−) process is clearly visible. This relaxation mechanism is the dielectric manifestation of the dynamic glass transition and appears as a step of strength Δ ɛ in the frequency dependence of the dielectric constant ɛ ′, that is, the real part of the complex dielectric function. The dielectric strength, linked in isothermal conditions to the mean square dipole moment [28] , provides a measure of the volume fraction of molecules relaxing on the time and length scale of the glass transition. During annealing at 423 K (≈ T g BULK +50 K), the dielectric strength of a film of thickness d =21 nm of PS97 (where M w =97 kg mol −1 ) capped between layers of aluminium (interfacial energy γ PS/Al =5.6 mJ m −2 ) decreased by almost 30%, whereas the electric capacitance in the absence of polarization contributions, C ∞ , increased by ∼ 3%. Because of the direct proportionality between C ∞ and d −1 , the higher value of capacitance measured on annealing indicates a small ( ∼ 3%) shrinkage of the film. At the chosen annealing temperature, τ α ∼ 10 μs and τ REP <1 s, although Δ ɛ is a function of the annealing time, decaying at much longer times. On a logarithmic scale, the reduction rate of Δ ɛ ( t ) remains constant till t on ≈2×10 3 s, where the decay speeds up by 60%, finally recovering its starting value after t off ≈3×10 4 s ( Fig. 1 ). For films of different thicknesses, we also found discontinuities at t on and t off in the time evolution of ζ (a parameter free from uncertainties in the film thickness or in the electrode surface) and C ∞ . The appearance of those discontinuities can be explained by the presence of two different adsorption rates, designated as 'low' and 'high', appearing as a logarithmic contribution (linear background in a representation of Δ ɛ versus log( t )) and an exponential decay of characteristic timescale t high . We were able to extract the traces of the higher rate process from Δ ɛ ( t ) ( Fig. 1 ), subtracting the linear contribution of Δ ɛ low ( t ) at Δ ɛ ( t < t on ). It was possible to fit the time evolution of Δ ɛ high ( t ) by a single exponential growth, in agreement with kinetic models previously identified in the increase of bound mass during an adsorption process [25] . 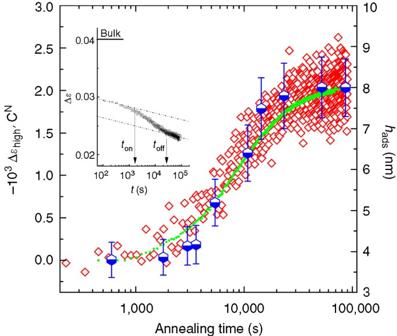Figure 1: Time evolution of the dielectric function in comparison with the growth of the adsorbed layer for PS97 during annealing at 423 K. Inset: the dielectric strength, Δɛ(black circles), of polymer nanocapacitors (aluminium/PS/aluminium) decreases on isothermal annealing atTg+50 K. For a 21-nm-thick film, the reduction rate of Δɛis constant at short timest<ton≈2×103s, where the decay speeds up by 60%, till finally recovering its starting value aftertoff≈3×104s. We extracted the traces of the higher rate process Δɛhigh(t) (red diamonds), subtracting the linear contribution at Δɛ(t<ton). The time evolution of Δɛhigh(t) matches the relative increase of the high frequency value of the capacitance,C∞(green dots, measured at 44 nm and normalized between the starting and final value of Δɛhighto ease comparison), and the growth of the thickness of the irreversibly adsorbed layer,hads, (semi open blue hexagons) in films annealed for different time at the same temperature of the isothermal experiments. Error bars forhadstake into account the uncertainties in the determination of film thickness from its geometrical capacitance, in the presence of an oxide layer on the aluminium surfaces. Figure 1: Time evolution of the dielectric function in comparison with the growth of the adsorbed layer for PS97 during annealing at 423 K. Inset: the dielectric strength, Δ ɛ (black circles), of polymer nanocapacitors (aluminium/PS/aluminium) decreases on isothermal annealing at T g +50 K. For a 21-nm-thick film, the reduction rate of Δ ɛ is constant at short times t < t on ≈2×10 3 s, where the decay speeds up by 60%, till finally recovering its starting value after t off ≈3×10 4 s. We extracted the traces of the higher rate process Δ ɛ high ( t ) (red diamonds), subtracting the linear contribution at Δ ɛ ( t < t on ). The time evolution of Δ ɛ high ( t ) matches the relative increase of the high frequency value of the capacitance, C ∞ (green dots, measured at 44 nm and normalized between the starting and final value of Δ ɛ high to ease comparison), and the growth of the thickness of the irreversibly adsorbed layer, h ads , (semi open blue hexagons) in films annealed for different time at the same temperature of the isothermal experiments. Error bars for h ads take into account the uncertainties in the determination of film thickness from its geometrical capacitance, in the presence of an oxide layer on the aluminium surfaces. Full size image Correlation between Δ ɛ and thickness of the Guiselin brushes To prove that the observed slow kinetics relates to the adsorption of polymer chains onto the solid surface, we reproduced Guiselin's experiment [29] and measured the thickness of the irreversibly adsorbed layer (Guiselin brushes) after annealing protocols performed under identical experimental conditions. The thickness of the Guiselin brushes, h ads , evolved with an exponential growth, h ads ( t ) ∼ 1−exp(− t / t ads ), from 3.8 to 8.0 nm ( Fig. 1 ). For films annealed at 423 K, the quantity of adsorbed chains remained constant for 2–3×10 3 s and then increased until reaching saturation at 3×10 4 s. The discontinuities related to the thickening of the adsorbed layer showed a clear correspondence with the changes in the time evolution of the dielectric spectra. We extended our experiments to different annealing temperatures and a different molecular weight. 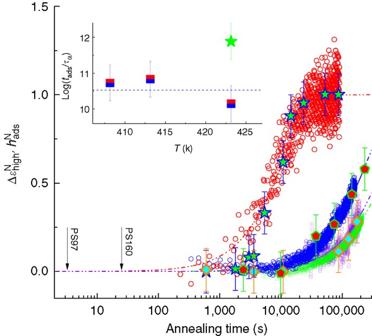Figure 2: Correlation between the time evolution of Δɛhighand the thickness of the adsorbed layer at different annealing temperatures and molecular weights. We extended experiments verifying that the correlation between the high rate component of the reduction of dielectric strength and the growth of the irreversibly adsorbed layer holds for different annealing temperatures and molecular weights. To facilitate comparison, we normalized each data set between the values assumed in the two plateau's (t<tonandt>toff); for those films in which the final plateau could not be reached during annealing, for the normalization we used the values obtained by fitting the traces of Δɛhigh(t) with an exponential decay (dash-dotted lines). Smaller symbols indicate Δɛhigh, whereas the thickness of the adsorbed layer is given by the larger symbols (PS97: 423 K red circles and blue/green stars, 413 K blue hexagons and green/red pentagons, 408 K violet pentagons; PS160: 423 K green squares and orange/cyan diamonds). Dot–dashed lines are fits of Δɛhigh(t) with an exponential function of the type Δɛhigh(t)=1−exp(−tads/t), wheretadsis time of the adsorption. For PS97 and PS160,tadsis more than 3 orders of magnitude longer than the reptation time (black arrows). In the inset: ratio betweentadsand the structural relaxation time,ταfor PS97 (red/blue squares) and PS160 (green star). Error bars are related to the experimental determination of the structural relaxation time by dielectric experiments. The results, summarized in Figure 2 , reveal a striking correlation between the growth of the Guiselin brushes and the impact of annealing on ultrathin films. The correlation established suggests equivalence between the characteristic time in the high rate component of the dielectric strength and the adsorption time, h ads ( t ) ∼ Δ ɛ high ( t ). Figure 2: Correlation between the time evolution of Δ ɛ high and the thickness of the adsorbed layer at different annealing temperatures and molecular weights. We extended experiments verifying that the correlation between the high rate component of the reduction of dielectric strength and the growth of the irreversibly adsorbed layer holds for different annealing temperatures and molecular weights. To facilitate comparison, we normalized each data set between the values assumed in the two plateau's ( t < t on and t > t off ); for those films in which the final plateau could not be reached during annealing, for the normalization we used the values obtained by fitting the traces of Δ ɛ high ( t ) with an exponential decay (dash-dotted lines). Smaller symbols indicate Δ ɛ high , whereas the thickness of the adsorbed layer is given by the larger symbols (PS97: 423 K red circles and blue/green stars, 413 K blue hexagons and green/red pentagons, 408 K violet pentagons; PS160: 423 K green squares and orange/cyan diamonds). Dot–dashed lines are fits of Δ ɛ high ( t ) with an exponential function of the type Δ ɛ high ( t )=1−exp(− t ads / t ), where t ads is time of the adsorption. For PS97 and PS160, t ads is more than 3 orders of magnitude longer than the reptation time (black arrows). In the inset: ratio between t ads and the structural relaxation time, τ α for PS97 (red/blue squares) and PS160 (green star). Error bars are related to the experimental determination of the structural relaxation time by dielectric experiments. Full size image For lower annealing temperatures and higher molecular weights, the adsorption kinetics slows down because of the less efficient transport of chains towards the interface. Such an increase in t ads cannot be explained in terms of bulk reptation [14] or 'sticky' reptation models [30] , which fail to describe the motion of polymer chains adsorbed on a solid substrate. Nevertheless, we were able to establish a criterion to predict the time and temperature effects of annealing on ultrathin films by comparing the temperature dependence of t ads with the relaxation times for segmental dynamics of bulk PS (inset of Fig. 2 ). In the temperature range investigated, the separation between the two processes (that is, the ratio between their characteristic timescales) remains constant, implying that the adsorption process and the dynamic glass transition have comparable activation energies. Similar analyses can be performed for the onset of the increase in the reduction rate of Δ ɛ , t on . In particular, for films of PS97 spincoated on aluminium, the adsorption process is 10–11 orders of magnitude slower than the α-relaxation, for example, at T g +50 K, annealing times longer than 10 4 τ REP are necessary to reach t off , whereas for PS160, this final time exceeds 6 weeks. Increasing M w by a factor smaller than 2 had the same impact on τ ads as a reduction of the annealing temperature by 15 K. Such a dependence of the adsorption kinetics on M w does not follow the scaling laws expected for the diffusion of the centre of mass of chains, probably because of chain pinning and a different interfacial entangling density [31] . These complications further retard the adsorption kinetics, and for M w above a critical value (for PS we expect for M w ∼ 300 kg mol −1 ), it is not possible to reach the condition t ann > t on on a laboratory timescale if the annealing temperature is kept out of the degradation regime. These conditions freeze the deviations from bulk behaviour of PS in metastable states with extremely long lifetimes. To achieve a deeper insight into the impact of those states on the properties of ultrathin films, we further analysed the mechanisms of adsorption of polymers from the melt onto a solid substrate. The non-zero thickness of the irreversibly adsorbed layer after short annealing above the bulk T g is in agreement with values of Δ ɛ ( t =0) smaller than Δ ɛ BULK by 20−30%, and with previous investigations [31] , [32] , [33] . Annealing, in fact, provokes the thickening of an adsorbed layer already formed during solvent evaporation and during the preannealing step, that is, already formed during the most commonly used annealing conditions. Adsorption begins with diffusion of chains towards the interface, in which the arriving molecules must find an empty space to stick. Partial or total immobilization of the chains limits the solid angle over which dipoles can reorient, yielding an effective lower mean square dipole moment and thus a lower dielectric strength. Macromolecules encounter a further complication: chains must explore different conformations in an attempt to minimize the free energy. This exploration happens via the formation of trains of segments interacting with the substrate, and it evolves with the collapse of the resulting loops, leading to a structural stabilization on increase of the segment/surface number [34] . The first logarithmic decay of the dielectric strength, characteristic of the latest stages of adsorption [31] , [35] , is the signature of these processes that probably begin even before reaching the measuring temperature. The presence of chains already adsorbed at the interface introduces a potential opposing insertion of new segments [35] and a bimodal energy landscape of the chain populations totally different from what is expected on the basis of a mere minimization of the free energy [32] . Although the first chains reaching the substrate spread over the available surface and absorb in relatively flat conformations, those arriving during later stages meet a more populated surface and can attach only by a reduced number of segments ( Fig. 3a–c ). The induction time before new segments can be absorbed ( ∼ t on ) scales with τ α and is limited by the constrained diffusion through the first incomplete layer [31] , [35] and the relaxation of those structures previously adsorbed, easing the insertion of new segments [32] , [36] . The final free energy balance is ruled by the enthalpic gain achieved by the formation of the adsorbed layer. Although driven by thermodynamic forces, the growth of the interfacial layer is a self-retarding process inhibited by the continuous reduction of the allowed conformations suitable for adsorption. These characteristics are reflected in the kinetics of Δ ɛ high ( t ), responsible for the irreversible physisorption of polymer segments onto the sites still available on the substrate at t > t on . Such a complex process, elegantly sketched by the idea of the 'lesser footprint' [32] , explains the extremely long times necessary to reach a steady state for the chain configurations of ultrathin polymer films and values of t on ≫ τ REP . We speculate that these mechanisms could be responsible for the unexpectedly long relaxation modes detected in other annealing experiments [15] , [16] , [17] , [18] , [19] , [20] . At t ∼ t off , the thickness of the residual layer doubles, and the probability of incorporating a larger quantity of chains is extremely low: a new metastable state, with a much longer lifetime, has been reached. 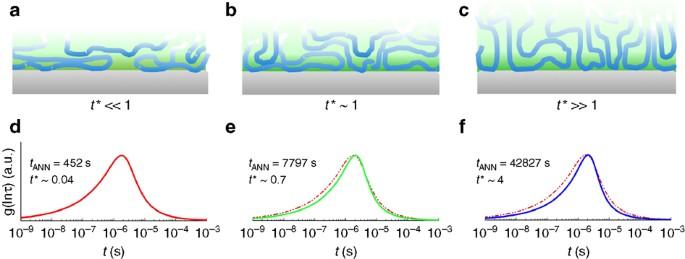Figure 3: Distribution of relaxation times and interfacial conformations. The impact of adsorption on the deviations from bulk behaviour can be rationalized in terms the dimensionless parametert*, corresponding to the ratio between the annealing and the adsorption time. The molecular picture corresponding to the perturbation in the dynamics on adsorption is given in (a–c). Up tot*∼1, adsorption proceeds via gradual filling of the available pinning sites at the interface, which provokes a decrease of the free volume in between molecules and causes the reduction in the population of faster modes. In the latest stages of adsorption,t*>1, the screening of previously adsorbed chains permits adsorption only on reorganization and pinning at fewer and fewer surface sites; the corresponding lower train fraction (percentage of sequences of consecutive monomers in direct contact with the surface) yields a reduction of the slower modes. Experimental validity of this molecular picture was achieved by analysing the distribution of relaxation times of the dielectric spectra of a 44-nm-thick film of PS97 during annealing at 423 K, at different adsorption conditions,t*=0.04 (d),t*=0.7 (e),t*=4 (f). Compared with short annealing times (t*≪1,d), adsorption induces a pronounced cutoff of the faster relaxation modes, after moderate annealing times (t*∼1,e). Further annealing (t*>1,f) induces a reduction in the polymer segments relaxing at slower characteristic times. Figure 3: Distribution of relaxation times and interfacial conformations. The impact of adsorption on the deviations from bulk behaviour can be rationalized in terms the dimensionless parameter t *, corresponding to the ratio between the annealing and the adsorption time. The molecular picture corresponding to the perturbation in the dynamics on adsorption is given in ( a – c ). Up to t * ∼ 1, adsorption proceeds via gradual filling of the available pinning sites at the interface, which provokes a decrease of the free volume in between molecules and causes the reduction in the population of faster modes. In the latest stages of adsorption, t *>1, the screening of previously adsorbed chains permits adsorption only on reorganization and pinning at fewer and fewer surface sites; the corresponding lower train fraction (percentage of sequences of consecutive monomers in direct contact with the surface) yields a reduction of the slower modes. Experimental validity of this molecular picture was achieved by analysing the distribution of relaxation times of the dielectric spectra of a 44-nm-thick film of PS97 during annealing at 423 K, at different adsorption conditions, t *=0.04 ( d ), t *=0.7 ( e ), t *=4 ( f ). Compared with short annealing times ( t * ≪ 1, d ), adsorption induces a pronounced cutoff of the faster relaxation modes, after moderate annealing times ( t * ∼ 1, e ). Further annealing ( t *>1, f ) induces a reduction in the polymer segments relaxing at slower characteristic times. Full size image Correlation between Δ T g and thickness of the adsorbed layer The conformations assumed by the chains in these states differ sensitively from those assumed by a polymer melt at conformational equilibrium, and they may thus induce different densities and different T g values. Although we are far from being able to determine more details of the energy landscape of those states, we want to stress the relevance of the correlations between the growth and relaxations of these interfacial layers and the changes in the performance of polymers in geometries with high surface-to-volume ratios. The link between the thickness of the residual layer and the drop in Δ ɛ high implies that thickening of the adsorbed layer proceeds mostly by an irreversible gradual filling of the empty spaces at the polymer/metal interface. In particular, the continuous thickening of the absorbed layer in the regime t on < t < t off provokes a reduction of the dynamic population of segments with dipoles reorienting faster than in bulk because of conformations eased by a larger local free volume ( Fig. 3a–c ). This idea is in line with the correlation between interfacial conformations and the T g in films of PMMA of different stereoregularity, spincast on Al (ref. 37 ). In the case of isotactic chains, a larger segment/surface ratio yields a higher interfacial T g , whereas lower transition temperatures are measured for syndiotactic PMMA, with a smaller number of bound segments per unit of area. With these considerations in mind, one might expect that, for a given isomer content, the glass-transition temperature during annealing evolves with the same kinetics as the formation of the irreversibly adsorbed layer and the correlated reduction in free volume at the interface, T g ( t ) ∼ h res ( t ). This picture is confirmed by the analysis of the distribution of relaxation times ( Fig. 3d–f ), where the suppression of the faster modes leads to an increase in τ α and consequently higher T g 's. It is then reasonable that these effects are comparable to the behaviour of a 'free surface' [5] , [38] , [39] that vanishes during annealing with the gradual anchoring of chains on the substrate and the consequent reduction of unoccupied sites at the interface. Our previous work on PS160 qualitatively supports this scenario [40] : the response of polymers annealed at lower temperatures mimic the trends of films with a layer of liquid-like thermal expansivity that does not vitrify when the system is cooled below bulk T g . Prolonged annealing was shown to remove the effects of the fast dynamics, increasing both the size of the immobilized layer and the value of T g . To quantitatively corroborate this physical picture, we measured, by means of capacitive dilatometry [41] , the T g 's of the Guiselin brushes of films of PS97 and of ultrathin films of PS97 and PS160 after different annealing times at 423 K. The shift in T g follows, as expected, the same kinetics as the irreversible adsorption process ( Fig. 4a,b ). 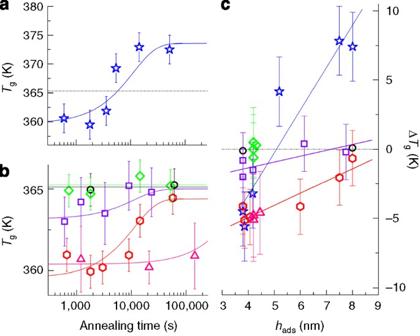Figure 4: Time evolution of the glass-transition temperature of films of PS97 and PS160 annealed for different times at 423 K. (a) The increase inTgof residual films of PS97 prepared at different annealing times follows the same kinetics as the irreversible adsorption process: the solid lines are obtained by normalization of the traces of Δɛhigh(t) collected during isothermal experiments. At short annealing times (t<ton),Tgis 5 K lower than in bulk (dash-dotted line) and increases till saturating atTgBULK+7 K att≫tads. (b) A similar correlation is observed for ultrathin films of different thickness and molecular weight: PS97, 18 nm (red hexagons), 35 nm (violet squares), 300 nm (black circles); PS160, 20 nm (pink triangles) and 44 nm (green diamonds). (c) The difference between theTgof the films (same symbols as ina,bwere used) and the bulk value, ΔTg, is plotted versus the thickness of the interfacial layer adsorbed in the same annealing conditions; straight lines are linear fits of the different data sets. Although for ultrathin films bulkTgis recovered att≫tads, for residual films of PS97 ΔTg=0 is achieved at much shorter times. Error bars take into account the width of the glass-transition temperature as determined by capacitive dilatometry in cooling. Figure 4c shows the corresponding direct proportionality between the thickness of the absorbed layers and the T g 's of the films, validating our hypothesis. In particular, following the traces of Δ ɛ high ( t ) for PS97, at short annealing times, the T g 's of the Guiselin brushes ( Fig. 4a ) and of films 18- and 35-nm thick ( Fig. 4b ) were, as expected, lower than the bulk (−5 and −2 K, respectively). After 20 h at 423 K, Δ T g (= T g (confined)− T g (bulk)) of the irreversibly adsorbed layer reached +8 K, whereas the T g of the thin films saturated at a temperature similar to the bulk value. Similar trends were found for films of PS160 ( Fig. 4b ), where the value of the reduced T g (−5 K) remained constant for longer times, reproducing the trend in the thickness of the adsorbed layer in Figure 2 . Thicker films (44 nm for PS160 and 300 nm PS97) showed no effect of annealing. Nevertheless, for films of 44 nm, we observed a variation of C ∞ ( t ) ∼ Δ ɛ high ( t ) ( Fig. 1 ), which can be explained by assuming that for d ≥35 nm, the error in the determination of T g is larger than the effective Δ T g . These last two results are in agreement with previous investigation of PS that showed no variation in T g (or Δ T g <2 K) above 40 nm or any impact of M w on T g ( d ) [42] . Figure 4: Time evolution of the glass-transition temperature of films of PS97 and PS160 annealed for different times at 423 K. ( a ) The increase in T g of residual films of PS97 prepared at different annealing times follows the same kinetics as the irreversible adsorption process: the solid lines are obtained by normalization of the traces of Δ ɛ high ( t ) collected during isothermal experiments. At short annealing times ( t < t on ), T g is 5 K lower than in bulk (dash-dotted line) and increases till saturating at T g BULK +7 K at t ≫ t ads . ( b ) A similar correlation is observed for ultrathin films of different thickness and molecular weight: PS97, 18 nm (red hexagons), 35 nm (violet squares), 300 nm (black circles); PS160, 20 nm (pink triangles) and 44 nm (green diamonds). ( c ) The difference between the T g of the films (same symbols as in a , b were used) and the bulk value, Δ T g , is plotted versus the thickness of the interfacial layer adsorbed in the same annealing conditions; straight lines are linear fits of the different data sets. Although for ultrathin films bulk T g is recovered at t ≫ t ads , for residual films of PS97 Δ T g =0 is achieved at much shorter times. Error bars take into account the width of the glass-transition temperature as determined by capacitive dilatometry in cooling. Full size image The trend in Figure 4 confirms that the dielectric strength is an adequate parameter for monitoring the effects of annealing in ultrathin polymer films. The time evolution of the glass-transition temperature could be reproduced by rescaling Δ ɛ high ( t ) between the values assumed in the two plateaus (continuous lines), which validate the relation T g ( t ) ∼ h ads ( t ) ∼ Δ ɛ high ( t ). On the basis of this equality, we can speculate that inhibiting or reducing adsorption ensures deviations from bulk behaviour with extremely long lifetimes (as for PS), a condition that can be quantified on the basis of the reduction in dielectric strength. The effects we described are not limited to the chains at the very interface. Several experimental observations have proven, in fact, that the influence of substrate interactions, which we can read here as the impact of adsorption, can propagate over hundreds of nanometres, in length scales proportional to the gyration radius of the polymer, R g . Although at early stages, only segments at the very interface are subjected to those conformational changes, prolonged annealing enables the adsorption of chains whose centre of mass lies in the core of the film [32] . In particular, chain pinning alters the surface dynamics of PS adsorbed on silicon (24 h at 443 K) up to thicknesses on the order of 4 R g and suppresses surface dynamics for layers thinner than R g [15] . Such a scaling is in line with our ideas on the impact of interfacial layers, as the thickness of the Guiselin brushes scales with R g itself [29] , [33] . Regardless of the extent of the distribution of conformations and the kinetics of adsorption, the trends in Figure 4 are in agreement with the idea that Δ T g is proportional to the polymer interface width [43] , that is, the thickness of the interfacial layer with non-bulk density. This final correlation, combined with the proportionality between t ads and τ α , suggests the feasibility of tuning the properties of polymers of conveniently low molecular weight confined in nanometre-thin films, of nanocomposites and of hybrid materials using moderate annealing, without altering the chemistry of the chains at the interface. Similarly, in the case of slow adsorption kinetics, for example, high M w 's, it is possible to freeze the value of T g in a steady state with extremely long lifetimes of months, years or perhaps longer. Finally, on the basis of the experimental evidence we introduced, it is convenient to introduce a non-dimensional parameter t *= t ANN / t ads , which, similarly to the Deborah number for viscoelasticity [44] , would link the deviations from bulk behaviour to the ratio of the timescale of adsorption (relaxation) to the annealing (observation) time. Provided that neither dewetting nor degradation nor crystallization occurs, for films annealed at t ann > t REP , we identify three regimes: (a) t * ≪ 1 ( t ≪ t on ), where chain adsorption is strongly limited by the hindrance of the existing incomplete first layer mimicking a free-surface effect, and chain rearrangements favouring adsorption could manifest as molecular processes with extremely long characteristic times; (b) t * ∼ 1 ( t on < t < t off ), where chains start to fill in the vacant sites on the substrate surface and undergo a series of metastable states and where confinement effects change continuously during the annealing time; and (c) t * ≫ 1 ( t ≫ t off ), where a new steady state is reached in which the solid surface is occupied by roughly a monolayer of strongly bound polymer coils (for PS on Al, h ads ∼ R g ). The properties of the new equilibrium are fixed by the boundary conditions imposed by the new interfacial configurations. The peculiar properties of these three regimes can explain the apparent contradictions in measurements performed under different annealing conditions. In particular, annealing protocols limited to a few reptation times correspond to the molecular weight-independent condition t * ≪ 1, justifying the lack of molecular weight dependence in the effects of thickness on the glass-transition temperature of supported and capped ultrathin films of PS. Preparation of polymer nanocapacitors for isothermal experiments Films of atactic PS of different molecular weights ( M w =97.4 kg mol −1 M w / M n =1.01, from Scientific Polymers, and M w =160 kg mol −1 M w / M n =1.06, from Pressure Chemical Company, indicated in the text as PS97 and PS160, respectively) were spincast from toluene (Acros 99+ extra pure % and Merck 99.9%, both HPLC grade) or chloroform (99.7% from Merck) directly onto thermally evaporated aluminium (Goodfellow 99%, evaporation rate ≥10 nm s −1 , thickness ∼ 50 nm; contact with air, before spincoating, favours the formation of a layer of 2–3 nm of oxide on top of the metal) and held for 2 h at 20 K above bulk T g (372±2 K from differential scanning calorimetry). Subsequently, samples were stored in a high vacuum chamber (pressure <10 −6 mbar) for more than 20 min (often left in vacuum overnight) to further reduce the amount of residual solvent. The preannealing conditions were chosen to allow release of stresses on timescales exceeding the reptation time ( t preann ≈24 τ REP PS97 ≈5 τ REP PS160 at 423 K) before starting isothermal experiments. Next, the upper surfaces of the films were metallized (Al, thermal evaporation in the same conditions described for the lower electrode) to permit the application of relatively low voltages to the resulting nanocapacitors. After evaporation of the upper electrode, samples were stored well below bulk T g until the isothermal measurements. By measuring the interfacial values of Δ ɛ and T g [21] , we verified that the impact of sample preparation on the two metal/polymer interfaces (spincoating polymer solutions on metal versus thermal evaporation on polymer surfaces) disappears after annealing for a short time (<15 min) at the same T ANN used in this work. Complex capacitances were measured using an impedance analyser (ALPHA, Novocontrol) under a continuous nitrogen flow. The thickness of the films ( d ) was measured by their geometrical capacitance at room temperature in an approximation of parallel plate geometry, which reads C ∞ = ɛ ∞ ɛ 0 (S/ d ), where C ∞ and ɛ ∞ indicate the capacitance of the film and the dielectric constant of the polymer (=2.5), respectively, in the absence of polarization processes, a condition reached at low temperatures ( T ≪ T g ) and high frequencies ( f >10 kHz); ɛ 0 indicates the vacuum permittivity (8.85×10 −12 F m −1 ); S indicates the surface area of the electrodes ( ∼ 4×10 −6 m 2 ) measured using optical microscopy; and d indicates the film thickness. The thickness of the polymer layers was also determined using ellipsometry. Following a procedure commonly used to reduce the number of fit parameters in the case of multilayers [2] , we determined the thickness of single polymer layers spincoated under the same experimental conditions used for the nanocapacitors (same solution, spinning and acceleration rate) on silicon oxide. The difference between the values obtained by the two independent methods was smaller than 2 nm. The small changes in film thickness during annealing (limited to 0.7 nm at 22 nm) disprove the occurrence of dewetting, which would cause larger fluctuations in the sample dimensions and thus in the electric capacitance. Moreover, in case of film rupture, direct contact between the metallic electrodes would cause a drop by more than 10 orders of magnitude in the electric impedance (shortcut), immediately recognizable in the dielectric spectra. We further verified using atomic force microscopy that the surface of films annealed more than 10 5 s presented no holes or other large thickness fluctuations that would indicate dewetting. To extract quantitative information from the isothermal dielectric spectra, relaxation processes were analysed using the empirical Havriliak–Negami (HN) function [45] where L ( τ ) is the distribution of relaxation times; Δ ɛ , τ HN , α , β are the dielectric strength, the relaxation time and the shape parameters, respectively, related to the width and the asymmetry of the loss curves. Integration of equation (1) permits the calculation of the distribution of relaxation times based on the fitting parameters of the HN-function. Preparation and characterization of the Guiselin brushes Shortly after spincasting, thick films ( ∼ 200–300 nm) deposited on thermally evaporated Al, were annealed for different times at the same temperature as the isothermal experiments. The non-adsorbed chains were washed away in the same good solvent used for spincoating (toluene) and dried in a vacuum ( P <10 −6 mbar) before evaporating a second layer of Al. The thickness of the adsorbed layers was calculated from their geometrical capacitance at room temperature. Corrections to the thickness of the polymer films considering the capacitive contribution of thin layer of aluminium oxide ( d ox =2–3 nm, ɛ ∞ =9.5) resulted in a small variation of h ads without altering the analytical form of h ads ( t ). Because of the higher dielectric constant, the contribution of aluminium oxide actually corresponds to that of an effective layer 3.8 (=9.5/2.5) times thinner, that is, 0.6−0.8 nm. The larger values of electric capacitance during annealing are not compatible with the idea of a growing oxide layer, as the sum of such a contribution (in a series model) would correspond to a reduction of the total capacitance. For films annealed at room temperature and washed in a good solvent, we obtained electrically shorted samples, implying the absence of an insulating polymer layer, that is, adsorption did not take place at thicknesses larger than the roughness of the electrodes (<2 nm). To facilitate comparison, we normalized each data set in Figure 2 between the values assumed in the two plateaus ( t < t on and t > t off ). For those films in which the final plateau could not be reached during annealing, we used the values obtained by fitting the traces of Δ ɛ high ( t ) with an exponential decay. Alternatively, normalization of the Guiselin brushes was also achieved by multiplying the thicknesses of the residual layers by a parameter a , typically on the order of 0.1–0.2 nm −1 , minimizing the expression . The traces of the higher rate process could also be fitted in terms of other analytical forms, such as, for example, the sum of a power law ( t < t off ) and a logarithmic contribution ( t > t off ), as proposed by Monte Carlo studies [31] . The choice of an exponential decay reduced the number of free parameters and provided a characteristic time for the process. Estimation of the interfacial energy between polymer and metal The interfacial energy γ PS/Al between aluminium and PS was calculated on the basis of the Good–Girifalco–Fowkes combining rule [46] , which takes into account both polar and dispersive contributions: where the superscripts LW, + and − indicate the dispersive, the electron acceptor (Lewis acid) and the electron donor (Lewis base) components, respectively, of the surface energy of either PS or Al. We used literature values for PS [47] , and we calculated the triad for Al [( γ LW =26.5, γ + =0.4, γ −=8.3) 10 −3 J m −2 ] from contact angle measurements on layers thermally evaporated under similar conditions performed in a previous work by one of the authors [48] . The contribution of the surface oxide layer to influencing the wettability of the metal is reflected in the values of the contact angle and is thus taken into account in the parameters of equation (2). The estimated interfacial energy (5.6 mJ m −2 ) is higher than the threshold value for PS (2 mJ m −2 ) [49] , indicating an attractive polymer/metal interaction and the onset of the reduction of segmental mobility in interfaces of PS. Determination of the glass-transition temperature Because of the direct proportionality between the capacitance of a dielectric medium and the inverse of its thickness, T g could be determined by the sudden reduction in thermal expansivity (here proportional to − dC ∞ /d T ) at the transition from the liquid to the glassy state [8] . Dielectric spectra were acquired under a continuous nitrogen flow with an effective cooling rate of −2 K min −1 . To inhibit further adsorption, measurements began at T ann −10 K. Because of the coupling with slower relaxation modes, T g determined by capacitive dilatometry is intrinsically lower (365±1 K for d >50 nm) than the transition temperature assigned in bulk by calorimetry, which instead coincide with the temperature where τ α is 100 s (373±1 K for d >100 nm) [21] . For PS, the thickness dependence of the T g of nanocapacitors determined by capacitive dilatometry is in line with experiments performed on supported films, via ellipsometry [50] . How to cite this article: Napolitano, S. & Wübbenhorst, M. The lifetime of the deviations from bulk behaviour in polymers confined at the nanoscale. Nat. Commun. 2:260 doi: 10.1038/ncomms1259 (2011).